YAP inhibits squamous transdifferentiation of Lkb1-deficient lung adenocarcinoma through ZEB2-dependent DNp63 repression Whether the Hippo pathway contributes to cell lineage transition under pathological conditions, especially tumorigenesis, remains largely unknown. Here we show that YAP, the major effector of the Hippo pathway, displays a distinct activation pattern in lung adenocarcinoma (ADC) and squamous cell carcinoma (SCC); YAP is initially activated by LKB1 loss in lung ADC, which upregulates ZEB2 expression and represses DNp63 transcription in a default manner. During transdifferentiation, YAP is inactivated, which in turn relieves ZEB2-mediated default repression of DNp63 and triggers squamous differentiation reprogramming. Disruption of the YAP barrier for phenotypic transition significantly accelerates squamous transdifferentiation, whereas constitutive YAP activation conversely inhibits this transition. More importantly, ectopic DNp63 expression rescues the inhibitory effect of YAP on squamous transdifferentiation. These findings have established YAP as an essential barrier for lung cancer cell fate conversion and provided a mechanism for regulating cancer plasticity, which might hold important implication for YAP-targeted therapies. The Hippo signalling pathway, initially identified in Drosophila , is a highly conserved and potent regulator of cell growth and apoptosis [1] , [2] . YAP is the main downstream effector of the Hippo pathway as a transcription cofactor and can be inactivated through its cytoplasmic retention and the phosphorylation by upstream kinases LATS1/2 (refs 3 , 4 ). Inactivation of the Hippo pathway leads to YAP nuclear translocation and downstream target genes expression by binding to the major transcription factor partner TEADs (the TEAD/TEF family transcription factors), resulting in cell survival and proliferation. Initially identified as an important regulator of organ size through the tight control of cell growth and proliferation, the Hippo pathway is now also considered to regulate cell fate determination, ranging from early embryonic development to adult tissue regeneration. YAP nuclear translocation and activation in polarized outer cells of embryo triggers TEADs-induced trophectoderm-specific transcriptional programme, whereas its cytoplasmic retention maintains the pluripotent status of the inner cell mass [5] , [6] , highlighting the activation of YAP as one of the first determining factors in guiding cell fate decision during early development. Moreover, YAP is also well documented to control the proliferation and lineage commitment of a wide spectrum of adult stem cells [4] , [7] , [8] , for example, YAP is shown to be an essential regulator of epidermal stem cell proliferation and expansion [9] . Mutations or epigenetic inactivation of upstream members of the Hippo pathway have been reported in different human malignancy [10] . YAP expression and nuclear localization are found to be elevated in human lung, colorectal, ovarian, liver and prostate cancers [11] , and significantly associated with poor prognosis [12] , [13] . In vitro and in vivo functional studies further highlight the oncogenic role of YAP in multiple organs through promoting cell proliferation, survival and neoplastic transformation [10] , [14] , [15] , [16] . Moreover, the contribution of YAP to cancer plasticity and cell fate determination began to emerge, for example, YAP promotes tumours to initiate the programme of epithelial–mesenchymal transition [10] . Our recent work has shown that Lkb1 inactivation confers lung adenocarcinoma (ADC) with strong plasticity and makes them progressively transit to squamous cell carcinoma (SCC) in mice [17] . This provides the first evidence to support the potential cell fate conversion implicated by the clinical observation of lung adenosquamous carcinoma (Ad-SCC), which contains mixed adenomatous and squamous pathologies with identical genetic alterations [18] . Lung ADC and SCC are two distinct lung cancer subtypes not only morphologically different but also featured with different gene expression signatures and cells of origin, for example, ADC is considered to arise mainly from alveolar epithelial cells such as type II pneumocytes with surfactant protein expression, whereas SCC is from basal cells with DNp63 expression [19] , [20] . Our findings about the transdifferentiation of mouse lung ADC to SCC highlight the existence of dynamic cell fate and lineage conversion in lung cancer progression. As YAP plays a crucial role in cell fate decision under physiological condition, it would be interesting to investigate the function of YAP in context with cell lineage transition accompanying tumour progression. Here we report YAP as a key player in cell-fate conversion during lung ADC to SCC transdifferentiation. Studies of mouse model and human clinical specimens identify a pathology-specific expression and distribution pattern of YAP. We further demonstrate that YAP acts as the important barrier for squamous transdifferentiation through DNp63 repression via transcriptional regulation of ZEB2 expression. Our findings shed light on the molecular basis for lung cancer phenotypic plasticity and provide important implications for YAP-targeted therapies in lung cancer. Differential YAP activation in lung ADC and SCC Our recent data show that lung ADC with Lkb1 deficiency can progressively transdifferentiate into SCC in Kras G12D , Lkb1 L/L ( KL ) mouse model [21] and all the SCC in this model are indeed derived from ADC [18] . Integrative bioinformatic analyses on microarray data sets derived from Lkb1-deficient mouse ADC and SCC have identified a series of significantly deregulated signalling pathways among which the Hippo pathway, previously shown to regulate cell fate determination during early embryonic development and adult tissue regeneration, caught our attention. Interestingly, we found a significantly different expression pattern of Yap target genes in these two distinct tumour subtypes: most of Yap target genes showed robust downregulation in SCC relative to ADC ( Fig. 1a ). Real-time PCR data further confirmed the decrease of most Yap target genes from 2- to 16-fold ( Fig. 1b ), implicating the differential YAP activities between ADC and SCC. Consistently, we observed a strong nuclear staining of Yap in ADC but low/no staining in SCC ( Fig. 1c ). Further real-time PCR analyses of clinical samples showed that most YAP target genes were dramatically decreased in SCC relative to ADC ( Fig. 1d ). More importantly, tissue microarray analyses demonstrated that the majority of SCC (62/84) exhibited low nuclear staining of YAP, whereas nearly half of ADC (37/83) had high nuclear YAP staining ( Fig. 1e ). 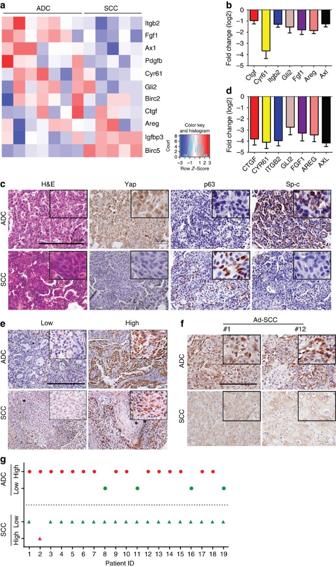Figure 1: Hippo pathway deregulation in ADC to SCC transdifferentiation. (a) Heat map showing significantly upregulated (red) and downregulated (blue) Yap target gene signatures between ADC and SCC fromKLmice. (b) Real-time PCR quantification of Yap target gene transcripts in ADC and SCC fromKLmice (each sample was assayed in triplicates). Fold change was calculated as log2 (SCC/ADC). (c) Representative images with haematoxylin and eosin staining, Yap, p63 and Sp-c immunohistochemical staining in ADC and SCC fromKLmice. Scale bar, 150 μm. (d) Real-time PCR quantification of YAP target gene transcripts in ADC and SCC from human lung cancer patients (each sample was assayed in triplicates). Fold change was calculated as log2 (SCC/ADC). (e) Representative images showing YAP immunohistochemical staining in ADC and SCC from human lung cancer patients. Scale bar, 150 μm. (f) Representative images showing YAP expression and subcellular location in human lung cancer samples with mixed histology of ADC and SCC. Scale bar, 150 μm. (g) YAP expression in the ADC and SCC portions from each mixed Ad-SCC samples. Paired Wilcoxon signed-rank test was used to determine the expression difference (Z=−3.742,P=0.000). Further cross-analyses of YAP expression and clinical pathological features revealed that YAP expression is significantly correlated with tumour pathologies ( Table 1 ). No correlation between LKB1 and YAP expression was found ( Supplementary Fig. 1 ). To explore the correlation between YAP expression and important human lung cancer oncogenotypes in ADC and SCC, we analysed multiple known oncogenic drivers, including EGFR , KRAS , HER2 and BRAF mutations, and EML4-ALK fusions in lung ADC and fibroblast growth factor receptor ( FGFR ) fusions in SCC, and performed clinical relevance analyses. Statistical analyses revealed a positive correlation between EGFR mutations and YAP expression ( Supplementary Table 1 ). 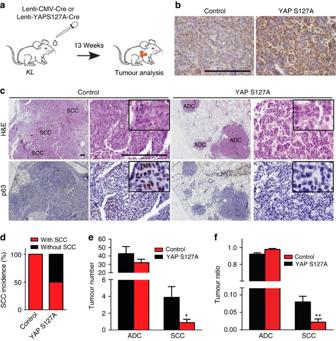Figure 2: Ectopic YAP expression inhibits ADC to SCC transdifferentiation. (a) Scheme of Lentivirus-mediated ectopic YAP S127A expression inKLmouse model. (b) YAP immunohistochemical staining in lung tumours fromKLmice delivered with Lenti-CMV-Cre or Lenti-YAPS127A-Cre. Scale bar, 150 μm. (c) Representative photos showing lung tumour formation and p63 immunohistochemical staining. Scale bar, 150 μm. (d) Quantification of SCC incidence ofKLmice delivered with Lenti-CMV-Cre (n=8) or Lenti-YAPS127A-Cre (n=8). (e,f) Quantification of average tumour number (e) and tumour ratio (f) per mouse for ADC and SCC fromKLmice delivered with Lenti-CMV-Cre (n=8) or Lenti-YAPS127A-Cre (n=8). Data are shown as mean±s.e.m.t-test, *P<0.05; **P<0.01. Moreover, we found that all the eight ADCs with EML4-ALK fusion exhibited low YAP expression ( Supplementary Table 2 ), indicating that this fusion and/or its downstream signalling might have compensatory function with YAP activation. 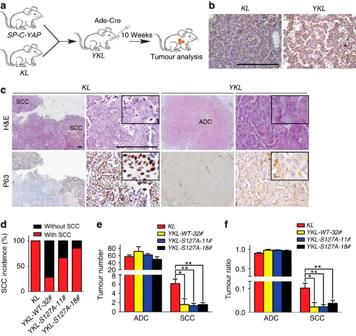Figure 3: Lineage-specific YAP expression inhibits ADC to SCC transdifferentiation. (a) Scheme of Ad-Cre treatment in establishedYKLmouse model. (b) Yap immunohistochemical staining in lung tumours fromKLorYKLmice at 10 weeks post Ad-Cre treatment. Scale bar, 150 μm. (c) Representative images for haematoxylin and eosin and p63 immunohistochemical staining inKLorYKLmice at 10 weeks post Ad-Cre treatment. Scale bar, 150 μm. (d) Quantification of SCC incidence ofKL(n=9) orYKLmice from threeSP-C-YAPtransgenic lines, includingYKL-WT-32#(n=7),YKL-S127A-11#(n=6) andYKL-S127A-18#(n=7). (e,f) Tumour number (e) and tumour ratio (f) quantification for ADC and SCC fromKL(n=9) orYKLmice from threeSP-C-YAPtransgenic lines, includingYKL-WT-32#(n=7),YKL-S127A-11#(n=6) andYKL-S127A-18#(n=7). Data are shown as mean±s.e.m.t-test, *P<0.05; **P<0.01. One YAP-positive SCC was found to have FGFR fusion ( Supplementary Table 3 ). We have also checked YAP expression and subcellular location in human lung Ad-SCC specimens with mixed histologies of ADC and SCC ( Fig. 1f,g ). Consistently, we found that the ADC part showed strong nuclear staining, whereas SCC did not ( Fig. 1f,g ). TAZ, the YAP paralogue that shares many transcription factor targets with YAP, is previously shown to contribute to lung cancer progression and metastasis [22] , [23] , [24] . However, unlike YAP, TAZ expression showed no significant correlation with lung cancer pathologies ( Supplementary Fig. 2 ). Collectively, our results uncovered the differential activation status of YAP in mouse and human lung cancer subtypes, suggesting a potential role of YAP in ADC and SCC cell-fate determination. Figure 1: Hippo pathway deregulation in ADC to SCC transdifferentiation. ( a ) Heat map showing significantly upregulated (red) and downregulated (blue) Yap target gene signatures between ADC and SCC from KL mice. ( b ) Real-time PCR quantification of Yap target gene transcripts in ADC and SCC from KL mice (each sample was assayed in triplicates). Fold change was calculated as log2 (SCC/ADC). ( c ) Representative images with haematoxylin and eosin staining, Yap, p63 and Sp-c immunohistochemical staining in ADC and SCC from KL mice. Scale bar, 150 μm. ( d ) Real-time PCR quantification of YAP target gene transcripts in ADC and SCC from human lung cancer patients (each sample was assayed in triplicates). Fold change was calculated as log2 (SCC/ADC). ( e ) Representative images showing YAP immunohistochemical staining in ADC and SCC from human lung cancer patients. Scale bar, 150 μm. ( f ) Representative images showing YAP expression and subcellular location in human lung cancer samples with mixed histology of ADC and SCC. Scale bar, 150 μm. ( g ) YAP expression in the ADC and SCC portions from each mixed Ad-SCC samples. Paired Wilcoxon signed-rank test was used to determine the expression difference ( Z =−3.742, P =0.000). Full size image Table 1 The clinical correlation of YAP expression in human NSCLC. Full size table YAP overexpression inhibits ADC to SCC transdifferentiation We then tested our hypothesis in de novo mouse model. We treated KL mice with 2 × 10 6 plaque forming unit (PFU) lentivirus carrying Cre recombinase with YAP S127A (a constitutively activated form of YAP) through nasal inhalation and confirmed its expression ( Fig. 2a,b and Supplementary Fig. 3a,b ). These mice were killed post 13 weeks of treatment for pathological analyses ( Fig. 2a ). As expected, all control KL mice (8/8) harboured both ADC and SCC ( Fig. 2c,d ). In contrast, only 50% (4/8) of mice in YAP S127A group developed SCC ( Fig. 2c,d ). Detailed analysis further supported that the number and ratio of SCC significantly decreased in YAP S127A group ( Fig. 2e,f ), indicating that forced YAP activation significantly suppressed the ADC to SCC transdifferentiation. Figure 2: Ectopic YAP expression inhibits ADC to SCC transdifferentiation. ( a ) Scheme of Lentivirus-mediated ectopic YAP S127A expression in KL mouse model. ( b ) YAP immunohistochemical staining in lung tumours from KL mice delivered with Lenti-CMV-Cre or Lenti-YAPS127A-Cre. Scale bar, 150 μm. ( c ) Representative photos showing lung tumour formation and p63 immunohistochemical staining. Scale bar, 150 μm. ( d ) Quantification of SCC incidence of KL mice delivered with Lenti-CMV-Cre ( n =8) or Lenti-YAPS127A-Cre ( n =8). ( e , f ) Quantification of average tumour number ( e ) and tumour ratio ( f ) per mouse for ADC and SCC from KL mice delivered with Lenti-CMV-Cre ( n =8) or Lenti-YAPS127A-Cre ( n =8). Data are shown as mean±s.e.m. t -test, * P <0.05; ** P <0.01. Full size image As lung ADC was mainly derived from type II pneumocytes, we took advantage of lineage-specific YAP expression to further study the role of YAP in lung cancer transdifferentiation. To this, we constructed two transgenic alleles expressing wide-type (WT) YAP or YAP S127A specifically in type II pneumocytes using SP-C promoter and crossed them with KL mice to obtain SP-C - Y AP WT/ S127A, K ras G12D , L kb1 L/L (YKL) mice. Both KL and YKL mice were analysed for YAP expression and detailed pathologies after 10 weeks of Adeno-Cre (Ad-Cre, 2 × 10 6 PFU) treatment ( Fig. 3a,b and Supplementary Fig. 3c,d ). Interestingly, we found that the penetrance of squamous transdifferentiation dramatically decreased in YKL mice derived from all three lines of SP-C - YAP WT/ S127A mice ( Fig. 3c,d ). The average SCC number and ratio also significantly decreased in YKL mice ( Fig. 3e,f ). These data together demonstrate that YAP overexpression suppresses the ADC to SCC transdifferentiation, indicating YAP as a potential barrier for this cell fate conversion. Figure 3: Lineage-specific YAP expression inhibits ADC to SCC transdifferentiation. ( a ) Scheme of Ad-Cre treatment in established YKL mouse model. ( b ) Yap immunohistochemical staining in lung tumours from KL or YKL mice at 10 weeks post Ad-Cre treatment. Scale bar, 150 μm. ( c ) Representative images for haematoxylin and eosin and p63 immunohistochemical staining in KL or YKL mice at 10 weeks post Ad-Cre treatment. Scale bar, 150 μm. ( d ) Quantification of SCC incidence of KL ( n =9) or YKL mice from three SP-C-YAP transgenic lines, including YKL-WT-32# ( n =7), YKL-S127A-11# ( n =6) and YKL-S127A-18# ( n =7). ( e , f ) Tumour number ( e ) and tumour ratio ( f ) quantification for ADC and SCC from KL ( n =9) or YKL mice from three SP-C-YAP transgenic lines, including YKL-WT-32# ( n =7), YKL-S127A-11# ( n =6) and YKL-S127A-18# ( n =7). Data are shown as mean±s.e.m. t -test, * P <0.05; ** P <0.01. Full size image Yap knockdown facilitates ADC to SCC transdifferentiation We next sought to explore whether YAP inactivation promotes the squamous transdifferentiation process. We delivered KL mice with lenti-U6-Cre (1 × 10 6 PFU) containing Yap short hairpin RNA (shRNA) and killed the mice post 18 weeks of treatment for pathological analyses ( Fig. 4a ). As expected, Yap knockdown led to a significant reduction of YAP expression ( Fig. 4b and Supplementary Fig. 4a ). We found a robust decrease of proliferating cells and a slight increase of cell apoptosis in lung ADC from shYap group ( Supplementary Fig. 4b,c ). This was further confirmed by in vitro data showing that YAP knockdown resulted in a significant decrease of A549 cell proliferation and anchorage-independent growth ( Supplementary Fig. 5a–c ). More importantly, Yap knockdown in KL mice significantly accelerated the squamous transdifferentiation ( Fig. 4c,d ). Consistently, the number and ratio of SCC but not ADC dramatically increased in shYap group ( Fig. 4e,f ). These data suggest that disruption of the barrier imposed by Yap significantly accelerates the ADC to SCC transdifferentiation. 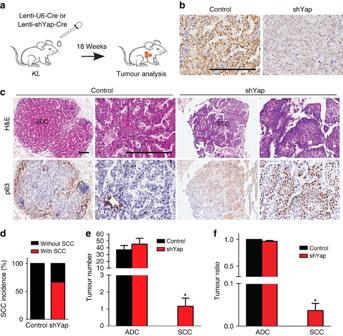Figure 4: Disruption of the YAP barrier for phenotypic transition significantly accelerates ADC to SCC transdifferentiation. (a) Scheme of Lentivirus-mediatedYapshRNA expression inKLmouse model. (b) YAP immunohistochemical staining in tumours fromKLmice delivered with Lenti-U6-Cre or Lenti-shYap-Cre. Scale bar, 150 μm. (c) Representative images with haematoxylin and eosin and p63 immunohistochemical staining in ADC and SCC fromKLmice delivered with Lenti-U6-Cre or Lenti-shYap-Cre. Scale bar, 150 μm. (d) Quantification of SCC incidence ofKLmice delivered with Lenti-U6-Cre (n=7) or Lenti-shYap-Cre (n=6). (e,f) Quantification of tumour number (e) and tumour ratio (f) for ADC and SCC fromKLmice delivered with Lenti-U6-Cre (n=7) or Lenti-shYap-Cre (n=6). Data are shown as mean±s.e.m.t-test, *P<0.05. Figure 4: Disruption of the YAP barrier for phenotypic transition significantly accelerates ADC to SCC transdifferentiation. ( a ) Scheme of Lentivirus-mediated Yap shRNA expression in KL mouse model. ( b ) YAP immunohistochemical staining in tumours from KL mice delivered with Lenti-U6-Cre or Lenti-sh Yap -Cre. Scale bar, 150 μm. ( c ) Representative images with haematoxylin and eosin and p63 immunohistochemical staining in ADC and SCC from KL mice delivered with Lenti-U6-Cre or Lenti- shYap -Cre. Scale bar, 150 μm. ( d ) Quantification of SCC incidence of KL mice delivered with Lenti-U6-Cre ( n =7) or Lenti- shYap -Cre ( n =6). ( e , f ) Quantification of tumour number ( e ) and tumour ratio ( f ) for ADC and SCC from KL mice delivered with Lenti-U6-Cre ( n =7) or Lenti- shYap -Cre ( n =6). Data are shown as mean±s.e.m. t -test, * P <0.05. Full size image Yap inhibits SCC transdifferentiation via DNp63 repression Surprisingly, we found that ~66.7% of mice from shYap group (4/6) harboured lung tumours with adenomatous pathology, but positive for p63 and Ck14 staining and negative for Sp-c staining ( Fig. 5a ), indicative of their transition status. This phenomenon was not detectable in control mice as well as KL mice with Ad-Cre treatment, suggesting the important role of Yap knockdown in promoting squamous transdifferentiation and maintaining the transition status. As YAP mainly functions as a transcriptional cofactor, we then asked whether YAP affects DNp63 expression at the transcriptional level. We found that ectopic YAP expression dramatically decreased DNp63 messenger RNA and protein level in human lung cancer cell lines HTB-182 and CRL-1848 ( Fig. 5b,c ). This regulation was also seen in a wide spectrum of lung cancer cell lines ( Supplementary Fig. 6a,b ). Conversely, YAP knockdown resulted in a significant increase of DNp63 mRNA and protein levels in multiple lung cancer cell lines, including HTB-182, CRL-1848 and A549 cells ( Fig. 5d,e and Supplementary Fig. 6c ). Constitutively active YAP mutant YAP-5SA strongly inhibited DNp63 transcription while this inhibitory effect was impaired in YAP 5SA-ΔC mutant with the deletion of its carboxy-terminal transactivation domain ( Fig. 5f,g and Supplementary Fig. 6d ), indicating YAP transcriptional activity is indispensible for DNp63 repression. 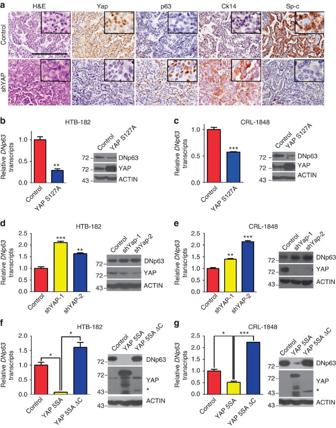Figure 5: YAP inhibits transdifferentiation through DNp63 repression. (a) Representative images showing haematoxylin and eosin and Yap, p63, Ck14 and Sp-c immunohistochemical staining on serial sections ofKLmice tumours delivered with Lenti-U6-Cre or Lenti-shYap-Cre. Scale bar, 150 μm. (b,c) Ectopic YAP S127A expression downregulated DNp63 mRNA and protein levels in HTB-182 (b) and CRL-1848 (c) cells. (d,e) Knockdown of YAP upregulated DNp63 mRNA and protein levels in HTB-182 (d) and CRL-1848 (e) cells. (f,g) Ectopic expression of YAP 5SA but not YAP 5SA with C-terminal transactivation domain deletion dramatically decreased DNp63 mRNA and protein levels in HTB-182 (f) and CRL-1848 (g) cells. The asterisk represents the YAP 5SA-ΔC mutant form with its C-terminal transactivation domain deletion. Each sample was assayed in triplicates by quantitative real-time PCR. Representative data of real-time PCR and western blotting were shown from three independent experiments. Data are shown as mean±s.e.m.t-test, *P<0.05; **P<0.01; ***P<0.005. Figure 5: YAP inhibits transdifferentiation through DNp63 repression. ( a ) Representative images showing haematoxylin and eosin and Yap, p63, Ck14 and Sp-c immunohistochemical staining on serial sections of KL mice tumours delivered with Lenti-U6-Cre or Lenti- shYap -Cre. Scale bar, 150 μm. ( b , c ) Ectopic YAP S127A expression downregulated DNp63 mRNA and protein levels in HTB-182 ( b ) and CRL-1848 ( c ) cells. ( d , e ) Knockdown of YAP upregulated DNp63 mRNA and protein levels in HTB-182 ( d ) and CRL-1848 ( e ) cells. ( f , g ) Ectopic expression of YAP 5SA but not YAP 5SA with C-terminal transactivation domain deletion dramatically decreased DNp63 mRNA and protein levels in HTB-182 ( f ) and CRL-1848 ( g ) cells. The asterisk represents the YAP 5SA-ΔC mutant form with its C-terminal transactivation domain deletion. Each sample was assayed in triplicates by quantitative real-time PCR. Representative data of real-time PCR and western blotting were shown from three independent experiments. Data are shown as mean±s.e.m. t -test, * P <0.05; ** P <0.01; *** P <0.005. Full size image Previous studies have implicated an essential role of extracellular matrix (ECM) in regulating YAP activity [25] , [26] , [27] , for example, cell detachment from ECM activates the Hippo pathway through cytoskeleton re-organization and leads to YAP phosphorylation and inactivation in immortalized human breast epithelial cells [27] . Our previous study identified a very distinct expression pattern of ECM components between ADC and SCC [17] . In an effort to investigate the potential involvement of ECM remodelling in modulating YAP activity and lung cancer transdifferentiation, we checked an expanded the list of genes involved in ECM remodelling (for example, collagen family and the collagen cross-linking key enzyme Lox family). Our data showed that most of these genes were robustly decreased in SCC relative to ADC ( Supplementary Fig. 7a ), consistent with our previous report [17] . We also found that ECM depletion by β-aminoproprionitrile (BAPN) treatment in KL mice significantly decreased the level of nuclear YAP in lung ADC ( Supplementary Fig. 7b ). Moreover, we found that cell detachment from ECM resulted in YAP phosphorylation and inactivation in A549 cells ( Supplementary Fig. 7c ). These data collectively provided evidences supporting that ECM deprivation in lung ADC might activate the Hippo pathway and lead to YAP phosphorylation and inactivation, which eventually induces DNp63 expression and initiates the squamous transdifferentiation programme. YAP represses DNp63 expression through ZEB2 To further explore the regulation of DNp63 by YAP, we initially investigated whether its major binding partners in the transcriptional complex, TEADs, mediated this process. Introduction of TEADs shRNA significantly reversed the downregulation of DNp63 expression by YAP 5SA ( Fig. 6a and Supplementary Fig. 6e ). As YAP-TEAD complexes usually activate downstream gene expression, we reasoned that YAP might repress DNp63 expression indirectly, through upregulating certain transcriptional repressors. We found six E-box sites from −2,229 to −237 bp upstream of DNp63 promoter, indicating the involvement of certain E-box-binding factors. We then screened the common E-box-binding factors, including SNAIL, SLUG, ZEB1, ZEB2 and MYC. Interestingly, ZEB2 turned out to be the only one consistently upregulated by YAP S127A in both A549 and HTB-182 cells ( Supplementary Fig. 8a,b ). We found that ectopic YAP S127A expression dramatically increased ZEB2 mRNA and protein levels in HTB-182, A549 and CRL-1848 cells ( Fig. 6b and Supplementary Fig. 9a,b ). Conversely, YAP knockdown significantly decreased ZEB2 mRNA and protein levels ( Fig. 6c and Supplementary Fig. 9c,d ). Moreover, our data showed that both YAP transactivation domain ( Fig. 6d and Supplementary Fig. 9e,f ) and TEADs ( Supplementary Fig. 9g ) were required for YAP transcriptional activation of ZEB2. We further identified a classical TEADs-binding site (GGAATG) at −557 bp upstream of the ZEB2 transcriptional start site. Reporter gene assay showed that ectopic YAP S127A expression increased ZEB2 promoter activity, while deletion of the TEADs-binding site attenuated the response of ZEB2 promoter to YAP S127A expression ( Fig. 6e ). Chromatin immunoprecipitation (ChIP) assay further confirmed the de novo binding of YAP to ZEB2 promoter region ( Fig. 6f ). 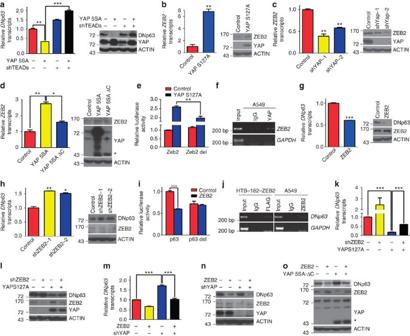Figure 6: YAP regulates DNp63 expression through ZEB2. (a) Knockdown of TEADs reversed the decrease of DNp63 mRNA and protein levels caused by YAP 5SA ectopic expression in HTB-182 cells. (b) YAP S127A ectopic expression upregulated ZEB2 mRNA and protein levels in HTB-182 cells. (c) YAP RNA interference (RNAi) downregulated ZEB2 mRNA and protein levels in HTB-182 cells. (d) Ectopic expression of YAP 5SA but not YAP 5SA with C-terminal transactivation domain deletion significantly increased ZEB2 mRNA and protein levels in HTB-182 cells. (e) YAP S127A ectopic expression significantly increased the transcriptional activity of ZEB2 wild-type promoter but not mutant with deletion of TEADs-binding site in 293T cells. (f) ChIP assay confirmed YAP binding to ZEB2 promoter in A549 cells. Glyceraldehyde 3-phosphate dehydrogenase (GAPDH) served as negative control. (g) ZEB2 ectopic expression downregulated DNp63 mRNA and protein levels in HTB-182 cells. (h) ZEB2 RNAi upregulated DNp63 mRNA and protein levels in HTB-182 cells. (i) ZEB2 overexpression decreased the transcriptional activity of DNp63 wild-type promoter but not mutant with deletion of ZEB2-binding site in L78 cells. (j) ChIP assay confirmed ZEB2 binding to DNp63 promoter in FLAG-ZEB2-transfected HTB-182 and A549 cells. GAPDH served as negative control. (k,l) Knockdown of ZEB2 reversed the decrease of DNp63 mRNA (k) and protein (l) levels caused by YAP ectopic expression in HTB-182 cells. (m,n) Re-introduction of ZEB2 abolished the increase of DNp63 mRNA (m) and protein (n) levels resulted from YAP knockdown in HTB-182 cells. (o) Re-introduction of ZEB2 abolished the increase of DNp63 protein levels caused by YAP 5SA-ΔC ectopic expression in HTB-182 cells. The asterisk represents the YAP 5SA-ΔC mutant form with its C-terminal transactivation domain deletion. Each sample was assayed in triplicates by quantitative real-time PCR and reporter gene assay. Representative data of real-time PCR, western blotting, ChIP and reporter gene assay were shown from three independent experiments. Data are shown as mean±s.e.m.t-test, *P<0.05; **P<0.01; ***P<0.005. Figure 6: YAP regulates DNp63 expression through ZEB2. ( a ) Knockdown of TEADs reversed the decrease of DNp63 mRNA and protein levels caused by YAP 5SA ectopic expression in HTB-182 cells. ( b ) YAP S127A ectopic expression upregulated ZEB2 mRNA and protein levels in HTB-182 cells. ( c ) YAP RNA interference (RNAi) downregulated ZEB2 mRNA and protein levels in HTB-182 cells. ( d ) Ectopic expression of YAP 5SA but not YAP 5SA with C-terminal transactivation domain deletion significantly increased ZEB2 mRNA and protein levels in HTB-182 cells. ( e ) YAP S127A ectopic expression significantly increased the transcriptional activity of ZEB2 wild-type promoter but not mutant with deletion of TEADs-binding site in 293T cells. ( f ) ChIP assay confirmed YAP binding to ZEB2 promoter in A549 cells. Glyceraldehyde 3-phosphate dehydrogenase (GAPDH) served as negative control. ( g ) ZEB2 ectopic expression downregulated DNp63 mRNA and protein levels in HTB-182 cells. ( h ) ZEB2 RNAi upregulated DNp63 mRNA and protein levels in HTB-182 cells. ( i ) ZEB2 overexpression decreased the transcriptional activity of DNp63 wild-type promoter but not mutant with deletion of ZEB2-binding site in L78 cells. ( j ) ChIP assay confirmed ZEB2 binding to DNp63 promoter in FLAG-ZEB2-transfected HTB-182 and A549 cells. GAPDH served as negative control. ( k , l ) Knockdown of ZEB2 reversed the decrease of DNp63 mRNA ( k ) and protein ( l ) levels caused by YAP ectopic expression in HTB-182 cells. ( m , n ) Re-introduction of ZEB2 abolished the increase of DNp63 mRNA ( m ) and protein ( n ) levels resulted from YAP knockdown in HTB-182 cells. ( o ) Re-introduction of ZEB2 abolished the increase of DNp63 protein levels caused by YAP 5SA-ΔC ectopic expression in HTB-182 cells. The asterisk represents the YAP 5SA-ΔC mutant form with its C-terminal transactivation domain deletion. Each sample was assayed in triplicates by quantitative real-time PCR and reporter gene assay. Representative data of real-time PCR, western blotting, ChIP and reporter gene assay were shown from three independent experiments. Data are shown as mean±s.e.m. t -test, * P <0.05; ** P <0.01; *** P <0.005. Full size image ZEB2 belongs to δEF-1 family of two-handed zinc finger transcription factors and generally functions as a DNA-binding transcriptional repressor [28] . We found ectopic ZEB2 expression significantly decreased DNp63 mRNA and protein levels in HTB-182, A549 and CRL-1848 cells ( Fig. 6g and Supplementary Fig. 10a,b ). Conversely, ZEB2 knockdown upregulated DNp63 transcription ( Fig. 6h and Supplementary Fig. 10c,d ). We then performed reporter gene assay using DNp63 proximal promoter region containing the ZEB2-binding site (−237 bp upstream of DNp63 transcriptional start site). ZEB2 expression dramatically reduced the activity of DNp63 promoter, which was abolished on deletion of ZEB2-binding site ( Fig. 6i ). We overexpressed ZEB2 in HTB-182 cells and confirmed its binding to DNp63 promoter through ChIP assay ( Fig. 6j ). Moreover, the de novo binding of ZEB2 to DNp63 promoter was also observed in A549 cells ( Fig. 6j ), indicating a novel default repression mechanism mediated by ZEB2 to keep DNp63 silent. We further found that ZEB2 knockdown rescued the inhibitory effect of YAP on DNp63 transcription ( Fig. 6k,l and Supplementary Fig. 11a,b ), while re-introduction of ZEB2 impaired the increase of DNp63 mRNA and protein level resulted from either YAP knockdown or deletion of the transactivation domain in HTB-182 cells ( Fig. 6m–o ). Similar results were also observed in A549 and CRL-1848 cells ( Supplementary Fig. 11c,d ). Taken together, these data supported the default repression of DNp63 expression by YAP in a ZEB2-dependent manner. DNp63 rescues squamous transdifferentiation inhibited by YAP We next explored the role of DNp63 in mediating YAP function during the ADC to SCC transdifferentiation using estrogen receptor (ER)-mediated DNp63-inducible expression [29] . We first confirmed that Tamoxifen (TAM) treatment increased nuclear DNp63 expression with a concomitant decrease of cytoplasmic DNp63 level as shown by western blotting using cytoplasmic and nuclear fractions ( Supplementary Fig. 12 ). We then treated YKL mice with Lenti-Cre expressing DNp63-ER through nasal inhalation, and 8 weeks later these mice were given TAM daily to induce DNp63 activation for another 4 weeks ( Fig. 7a ). In stark contrast, TAM-treated mice showed strong evidences for squamous transdifferentiation, whereas no detectable p63-positive SCC lesions were observed in control mice ( Fig. 7b,c ). The average SCC number and ratio were also increased in TAM treatment group ( Fig. 7d,e ). These data demonstrated that DNp63 overexpression overcome the barrier of squamous transdifferentiation imposed by YAP, further highlighting the central role of DNp63 in initiation of squamous reprogramming downstream of YAP. 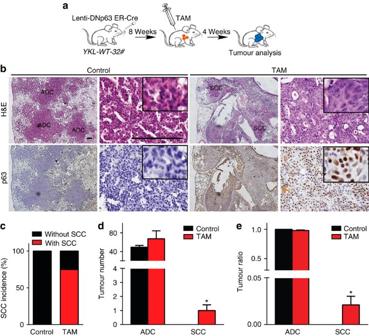Figure 7: DNp63 rescues the inhibitory effect of YAP on SCC transdifferentiation. (a) Scheme of ER-inducible DNp63 expression strategy inYKL-WT-32#mice. (b) Representative photos for haematoxylin and eosin and p63 immunohistochemical staining inYKLmice treated with TAM or sunflower oil after Lenti-DNp63 ER-Cre infection. Scale bar, 150 μm. (c) Quantification of SCC incidence ofYKL-WT-32#mice treated with TAM (n=4) or sunflower oil (n=4) after Lenti-DNp63 ER-Cre infection. (d,e) Quantification of tumour number (d) and tumour ratio (e) for ADC and SCC fromYKL-WT-32#mice treated with TAM (n=4) or sunflower oil (n=4) after Lenti-DNp63 ER-Cre infection. Data are shown as mean±s.e.m.t-test, *P<0.05. Figure 7: DNp63 rescues the inhibitory effect of YAP on SCC transdifferentiation. ( a ) Scheme of ER-inducible DNp63 expression strategy in YKL-WT-32# mice. ( b ) Representative photos for haematoxylin and eosin and p63 immunohistochemical staining in YKL mice treated with TAM or sunflower oil after Lenti-DNp63 ER-Cre infection. Scale bar, 150 μm. ( c ) Quantification of SCC incidence of YKL-WT-32# mice treated with TAM ( n =4) or sunflower oil ( n =4) after Lenti-DNp63 ER-Cre infection. ( d , e ) Quantification of tumour number ( d ) and tumour ratio ( e ) for ADC and SCC from YKL-WT-32# mice treated with TAM ( n =4) or sunflower oil ( n =4) after Lenti-DNp63 ER-Cre infection. Data are shown as mean±s.e.m. t -test, * P <0.05. Full size image YAP/ZEB2 negatively correlates with p63 expression in lung cancer We further tested whether the regulation of p63 by YAP/ZEB2 signalling axis existed in de novo lung cancer progression and transdifferentiation process. Indeed, we found a marked induction of ZEB2 expression in mouse lung tumours with ectopic YAP S127A expression ( Fig. 8a ); conversely, a dramatic decrease of ZEB2 expression in lung tumours was seen when shYap was introduced to KL mice ( Fig. 8b ). Moreover, the inverse correlation between ZEB2 and p63 expression was consistently observed in lung tumours from KL mice ( Fig. 8c and Supplementary Table 4 ). 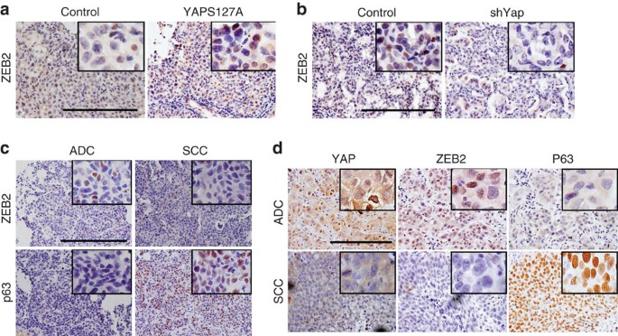Figure 8: YAP/ZEB2 reversely correlate with p63 expression in lung cancer. (a) ZEB2 immunohistochemical staining in lung tumours fromKLmice delivered with Lenti-CMV-Cre or Lenti-YAPS127A-Cre. Scale bar, 150 μm. (b) ZEB2 immunohistochemical staining in tumours fromKLmice delivered with Lenti-U6-Cre or Lenti-shYap-Cre. Scale bar, 150 μm. (c) Representative photos showing ZEB2 and p63 immunohistochemical staining on serial sections of ADC and SCC tumours fromKLmice. Scale bar, 150 μm. (d) Representative photos showing YAP, ZEB2 and p63 immunohistochemical staining in ADC and SCC from human lung cancer patients. Scale bar, 150 μm. Figure 8: YAP/ZEB2 reversely correlate with p63 expression in lung cancer. ( a ) ZEB2 immunohistochemical staining in lung tumours from KL mice delivered with Lenti-CMV-Cre or Lenti-YAPS127A-Cre. Scale bar, 150 μm. ( b ) ZEB2 immunohistochemical staining in tumours from KL mice delivered with Lenti-U6-Cre or Lenti- shYap -Cre. Scale bar, 150 μm. ( c ) Representative photos showing ZEB2 and p63 immunohistochemical staining on serial sections of ADC and SCC tumours from KL mice. Scale bar, 150 μm. ( d ) Representative photos showing YAP, ZEB2 and p63 immunohistochemical staining in ADC and SCC from human lung cancer patients. Scale bar, 150 μm. Full size image We further conducted tissue array analyses focusing on YAP, ZEB2 and p63 expression pattern to explore the potential clinical relevance of our findings in animal models. Notably, YAP and ZEB2 exhibited high nuclear expression in ADC but low or diffused cytoplasmic staining in SCC, which were negatively associated with p63 expression ( Fig. 8d ). Correlation analyses showed that ZEB2 expression positively correlated with YAP expression while negatively correlated with p63 expression in human lung cancer samples ( Table 2 ). Collectively, our findings uncovered a key role of YAP/ZEB2/p63 signalling axis in lung ADC to SCC transdifferentiation and provided novel mechanistic insights into the cell-fate determination in human malignancy. Table 2 Expression correlation between YAP, ZEB2 and p63 in human NSCLC. Full size table It is now well established that the cells of origin and acquired gene mutations act in concert to control tumour histopathology and phenotype [30] , [31] . Lineage tracing studies in Genetically Engineered Mouse Models have uncovered the existence of tumour cell lineage transition during tumorigenesis, leading to drug resistance and growth advantage to promote malignant progression [30] , [31] . Glioblastoma stem cells could give rise to endothelial cells to facilitate tumour angiogenesis [32] , [33] . Nkx2-1 deletion promotes lung ADC to transdifferentiate towards gastric lineage [34] . Consistently, clinical studies have found convergent mutations in both ADC and SCC components from a single lesion of human Ad-SCC [35] , [36] , [37] , [38] , [39] , leading to the hypothesis that there exists dynamic cell lineage conversion between these two pathologically and morphologically distinct tumour subtypes. Our work in Lkb1-deficient mouse models has recently provided the first de novo evidences supporting this hypothesis [18] . It is worth noting that the ADC to SCC transdifferentiation is unlikely related to the classical cancer stem cell theory, in which only a small population of cancer cells were endowed with strong plasticity [32] , [33] . Indeed, multiple lines of evidences from previous study have supported that the majority, if not all, of lung ADC cells with Lkb1 deficiency are capable to transit to SCC [17] . As the Hippo signalling is actively involved in cell-fate determination from early embryonic development to adult tissue homeostasis, we speculate that YAP might potentially contribute to cell lineage transition and regulate cancer phenotypic plasticity. Our work here indeed establishes an essential role of YAP in inhibiting lung ADC to SCC transdifferentiation. With integrative studies of mouse models, human lung cancer cell lines and clinical specimens, we prove that ectopic YAP expression dramatically suppresses squamous transdifferentiation while YAP knockdown accelerates this process. These findings identify YAP as an important barrier for lineage conversion during lung cancer transdifferentiation process and link the lineage-restricted signalling, which normally operates during embryonic development, to cell-fate transition accompanying cancer progression. We further identify an unexpected regulation of DNp63 by YAP. Mounting evidences have supported DNp63 as an important lineage survival oncogene in SCC from multiple tissues [40] , [41] . Our findings here demonstrate that DNp63 induction triggered by YAP downregulation in lung ADC is a critical step in the systematic squamous reprogramming. YAP activation in lung ADC induces ZEB2 expression, and the latter binds to DNp63 gene promoter and represses DNp63 transcription. During the squamous transdifferentiation process, YAP downregulation relieves ZEB2-mediated default repression on DNp63 transcription, leading to the initiation of squamous reprogramming. Our findings indicate that dysregulation of DNp63 triggered by YAP inactivation is functionally related to lung cancer transdifferentiation in the context of LKB1 mutant ADC and Ad-SCC with mixed pathologies. Previous study has shown that YAP can bind to and stabilize p63 in keratinocytes to protect damage from ultraviolet irradiation [42] . Interestingly, we find that YAP and DNp63 show a reverse correlation in lung ADC and SCC, which might be resulted from the default transcriptional repression of DNp63 by YAP. This represents a new tissue-specific regulatory pattern between YAP and DNp63. A recent study reports ZEB1 dynamically controls breast cancer cell plasticity through chromatin configuration in response to environmental stimuli [43] . Despite of a slight upregulation of ZEB1 by YAP, the regulation of ZEB2 seems more dramatic and consistent in our study. Our data further support that ZEB2 is indeed involved in the regulation of DNp63 by YAP. More importantly, this regulation seems consistent in mouse and human. Our functional data further demonstrate that ectopic DNp63 expression rescues the inhibitory effect of YAP on SCC transdifferentiation, indicating its central role in squamous differentiation reprogramming elicited by YAP inactivation. Thus, the findings of YAP/ZEB2/DNp63 regulatory axis provide a novel mechanistic insight into lung cancer phenotypic plasticity and cell-fate determination during tumour progression. YAP is frequently activated in various epithelial cancer types and considered as a rising star for cancer therapeutics [10] . Nonetheless, several other studies also implicate YAP as a tumour suppressor [44] , [45] , [46] , suggesting that YAP might have opposing functions in organ- and genetic-context-dependent manner. Our data have shown that YAP knockdown in A549 cells resulted in decreased cell proliferation and anchorage-independent cell growth in vitro ( Supplementary Fig. 5 ). Moreover, Yap knockdown in KL mice results in a robust decrease of proliferating cells and a slight increase of cell apoptosis in lung ADC ( Supplementary Fig. 4 ). These data suggests YAP might serve as an attractive therapeutic target for lung ADC with LKB1 deficiency, which represents a unique and prevalent molecular subtype of lung cancer with few effective treatments available. However, our findings here also raise some concerns towards targeting YAP in consideration of the differential expression and function of YAP in distinct tumour pathologies. YAP activity is surprisingly low in lung SCC relative to ADC in both mouse and human specimens. Moreover, YAP inactivation promotes cell-fate conversion and tumour subtype transition. Our previous report shows that ADC and SCC might display different response towards certain therapies [17] . Thus, the cell-fate transition might represent a mechanism for lung ADC developing resistance towards YAP-targeted therapy. In line with this, multiple reports also show that a phenotypic transition from ADC to small cell lung carcinoma (SCLC) promotes the drug resistance to EGFR tyrosine kinase inhibitors [47] , [48] . For these complicate diseases, tumour-type-specific and/or combinatory targeting strategies might be required to achieve more effective clinical outcomes for YAP-targeted therapy, especially to LKB1-mutant lung cancer. Our findings about the fundamental role of YAP in regulating lung cancer lineage conversion and phenotypic transition might help future development of better therapeutic strategies. Human lung cancer specimen collection All the human lung ADC and SCC specimens were collected in Fudan University Shanghai Cancer Center from November 2007 to July 2010, with patient written consents and the approval from the Institute Research Ethics Committee. All tumour specimens were taken at the time of surgical resection. Clinical–pathologic features, including age at diagnosis, gender, smoking history, histology, stage and tumour differentiation status, were collected. Eighty-two lung ADC samples, 84 SCC and 19 mixed Ad-SCC samples were used for immunohistochemistry analysis. Ten lung ADC specimens and nine SCC specimens were used for real-time PCR analyses. Mouse cohorts and treatment All mice were housed in a specific pathogen-free environment at the Shanghai Institute of Biochemistry and Cell Biology and treated in strict accordance with protocols approved by the Institutional Animal Care and Use Committee of the Shanghai Institutes for Biological Sciences, Chinese Academy of Sciences. Kras G12D and Lkb1 L/L mice were originally generously provided by Dr T. Jacks and Dr R. Depinho, respectively. To generate the SP-C-YAP WT and SP-C-YAP S127A transgenic mice, a DNA fragment with human YAP WT and S127A coding region and SV40 poly A was ligated to the human SP-C promoter and microinjected into C57 blastocysts. Progeny were screened by Southern blotting and confirmed by PCR strategy. KL and YKL mice (male and female at 8 weeks of age) were treated with Ad-Cre (2 × 10 6 PFU). Mice were then killed at 10 weeks post Ad-Cre nasal inhalation. KL mice (male and female at 8 weeks of age) were treated with lenti-YAP S127A-Cre (2 × 10 6 PFU) or lenti-sh Yap -Cre (1 × 10 6 PFU) via nasal inhalation. Next, mice were killed at 13 and 18 weeks, respectively. For YKL mice (male at 8 weeks of age) treated with 2 × 10 6 PFU lentivirus (lenti-DNp63-ER-Cre), TAM diluted in sunflower oil (40 mg kg −1 ) were given to mice via intraperitoneal injection 8 weeks post lentivirus administration, and YKL mice were killed following 4 weeks TAM daily administration. Histopathological analysis All mice were killed for gross inspection and histopathological examination. Mice lung tissues were inflated and fixed in 4% formalin, embedded in paraffin, sectioned and stained with haematoxylin and eosin. Histological examinations were performed by a pathologist and tumour number was counted under microscope. Tumours on mice lung surface were dissected and collected for molecular analysis. Cell culture, transfection and lentiviral infection NSCLC cell lines A549, CRL-5908, CRL-5807, CRL-5810, L78 and HTB-182, which were purchased from ATCC, were grown in RPMI 1640 medium supplemented with 10% fetal bovine serum (FBS). SH-416 was cultured in ACL4 plus 5% FBS. HEK-293T and CRL-1848 were cultured in DMEM containing 10% FBS. Lentiviral infection was done as follows: HEK-293T cells were co-transfected with pLKO.1 or pCDH constructs and packaging plasmids. The medium containing progeny virus released from HEK-293T cells were filtered, collected and used to infect NSCLC cells. Cell proliferation and anchorage-independent cell growth For cell proliferation assay, cells were seeded on 96-well plates and the viability of cells was measured by MTT (3-(4,5-dimethylthiazol-2-yl)-2,5-diphenyltetrazolium bromide) assay daily for 5 days. Anchorage-independent cell growth was assessed by soft agar assay. Briefly, 5,000 viral-infected cells were suspended in growth medium with 0.4% agar on top of 1% agar base in six-well plates. After 2 weeks culture, colonies were stained with 0.005% crystal violet and counted by Image-J. All experiments were performed in triplicates. RT–PCR and quantitative real-time PCR Total RNA was extracted using Trizol reagent (Invitrogen) and phenol/chloroform methods. RNA was retro-transcribed into first-strand complementary DNA using RevertAid First Strand cDNA Synthesis Kit (Fermentas). cDNAs were subjected to quantitative real-time PCR with gene-specific primers on 7,500 Fast Real-Time PCR System (Applied Biosystems) using SYBR-Green Master PCR mix (Invitrogen). Sequences of real-time PCR primers are listed in Supplementary Table 5 . Glyceraldehyde 3-phosphate dehydrogenase (human) or Actin (mouse) served as internal control. Luciferase reporter assay HEK-293T and L78 cells were seeded in 24-well plates. Luciferase reporter and indicated plasmids were co-transfected. Twenty-four hours after transfection, cells were lysed and luciferase activities were measured using Dual-Luciferase Assay kit (Promega) on GloMax 20/20 luminometer (Promega) following the manufacturer’s instructions. pRL-TK or pEGFP-N1 was co-transfected as internal control. Experiments were done in triplicates. Chromatin immunoprecipitation Cells were cross-linked, lysed and sonicated to generate DNA fragments with an average size of 500 bp. Two-microgram antibodies against YAP, ZEB2, Flag or control IgG were added to cell lysate. An aliquot of ChIP-enriched DNA and whole-cell lysate DNA were subjected to PCR using ChIP-specific primers listed in Supplementary Table 5 . Original pictures of gels are shown in Supplementary Fig. 13 . Immunohistochemical analysis Paraffin-embedded lung tissues were incubated with following antibodies: anti-YAP (Santa Cruz, sc-15407, 1:500 dilution; Cell Signaling Technologies, 4912, 1:500 dilution), anti-DNp63 (4A4) (Santa Cruz, sc-8431, 1:500 dilution), anti-ZEB2 (Abcam, ab25837, 1:500 dilution), anti-SP-C (Chemicon, AB3786, 1:2,500), anti-CK14 (Covance, PRB-155P, 1:1,000 dilution), anti-TAZ (Santa Cruz, sc-48805, 1:200) anti-LKB1 (Cell Signaling Technologies, 13031, 1:300 dilution), anti-Ki-67 (Novocastra, NCL-Ki67P, 1:500) and anti-Cleaved Caspase-3 (Cell Signaling Technologies, 9661, 1:800). Immunohistochemical scoring of YAP, ZEB2, TAZ and DNp63 expression was performed as follows: strong nuclear expression of the above genes in over 50% of the tumour cells was scored as high; cytoplasmic expression and nuclear expression in <50% of the tumour cells were scored as low. LKB1 immunoreactivity evaluation was carried out as follows: strong and uniform expression in over 10% of the tumour cells was scored as high; weak expression or strong expression in <10% of the tumour cells were scored as low. Nuclear and cytoplasmic protein extraction Preparation of nuclear and cytoplasmic extract was performed following manufacturer’s instructions (Beyotime Nuclear and Cytoplasmic Protein Extraction Kit). Cells were harvested by adding 0.125% trypsin-EDTA and lysated in buffer A on ice for 15 min and centrifuged at 16,000 g for 5 min. The supernatant containing the cytoplasmic proteins was removed and stored for use. The pellet was resuspended in buffer B. After incubation on ice for 30 min, lysates were centrifuged at 16,000 g for 15 min and the supernatants containing the nuclear proteins were stored for use. Immunoblotting Cells were lysed in lysis buffer and subjected to western blot analysis with following primary antibodies: anti-YAP (Santa Cruz, sc-15407, 1:500 dilution), anti-p-YAP (Cell Signaling Technologies, 4911, 1:1,000 dilution), anti-DNp63 (4A4) (Santa Cruz, sc-8431, 1:500 dilution), anti-ZEB2 (Abcam, ab25837, 1:500 dilution), anti-ACTIN (Sigma, A2228, 1:5,000 dilution), anti-LAMIN B (Santa Cruz, sc-6216, 1:1,000 dilution), anti-TUBULIN (Sigma, T5168, 1:2,000 dilution) and anti-glyceraldehyde 3-phosphate dehydrogenase (Abmart, M20006, 1:5,000 dilution). Original pictures of western blotting are shown in Supplementary Figs 13 and 14 . Plasmid construction The human TEAD1/3/4 shRNA construct is kindly provided by Professor Qunying Lei; the human YAP shRNA construct is generously given by Professor Zengqiang Yuan and the human ZEB2 expression vector is a gift from Professor Gaoxiang Ge. To generate YAP expression vectors, YAP S127A, YAP 5SA and YAP 5SA-ΔC were amplified from pQCXIH-based vectors [49] and inserted in frame into pCDH-CMV-EF1-Puro (Systems Biosciences). The open reading frame of YAP S127A and ER-fused DNp63 were also subcloned to pCDH-CMV-EF1-Cre vector (adapted vector for gene expression in vivo ). The shRNA towards mouse Yap was cloned to pCDH-U6-EF1-Cre vector (adapted vector for gene knockdown in vivo ). The ZEB2 1,107-bp and DNp63 350-bp promoters were cloned from human genomic DNA into the pGL3-Basic vector. The binding-site mutants were generated by deletion of 5′-CCTTAC-3′ in Zeb2 promoter and 5′-CAGGTG-3′ in DNp63 promoter. The shRNAs towards human ZEB2 and mouse Yap were cloned into pLKO.1 (Addgene) with the Age I/ Eco RI sites. The target sequences are as follows. shYap : 5′-UGAGAACAAUGACAACCAAUA-3′ shZEB2 -1: 5′-CCACUAGACUUCAAUGACUAU-3′ shZEB2 -2: 5′-CCACAACAUAUCCACUCCAUU-3′ Bioinformatic analysis We used the public GSE6135 data set containing mouse ADC and SCC for lung genes expression profiling. Robust multi-array average (RMA) normalization was applied to normalize expression of microarray samples. Custom Chip Definition Files of REFSEQ gene from Brainarray was used to match the individual probes ( http://brainarray.mbni.med.umich.edu/brainarray/default.asp ). All the expression samples were first transformed in to log2 scale and then normalized by quantile normalization. Heatmap figures were generated according to the expression profiles of the genes by the function heatmap.2 in R. The genes were ranked by the T -statistics of the T -test. Statistical analysis Data were represented as mean±s.e.m. and analysed by Student’s t -test (two-tailed). The χ 2 -test and Fisher’s exact test ( n <5) were used to determine the correlation between YAP expression and clinicopathologic factors. Paired Wilcoxon signed-rank test was used to determine YAP expression differences between ADC and SCC portions in mixed Ad-SCC samples. Differences with a P <0.05 were considered statistically significant. How to cite this article: Gao, Y. et al . YAP inhibits squamous transdifferentiation of Lkb1-deficient lung adenocarcinoma through ZEB2-dependent DNp63 repression. Nat. Commun. 5:4629 doi: 10.1038/ncomms5629 (2014).